Germinal centre protein HGAL promotes lymphoid hyperplasia and amyloidosis via BCR-mediated Syk activation The human germinal centre-associated lymphoma gene is specifically expressed in germinal centre B-lymphocytes and germinal centre-derived B-cell lymphomas, but its function is largely unknown. Here we demonstrate that human germinal centre-associated lymphoma directly binds to Syk in B cells, increases its kinase activity on B-cell receptor stimulation and leads to enhanced activation of Syk downstream effectors. To further investigate these findings in vivo , human germinal centre-associated lymphoma transgenic mice were generated. Starting from 12 months of age these mice developed polyclonal B-cell lymphoid hyperplasia, hypergammaglobulinemia and systemic reactive amyloid A (AA) amyloidosis, leading to shortened survival. The lymphoid hyperplasia in the human germinal centre-associated lymphoma transgenic mice are likely attributable to enhanced B-cell receptor signalling as shown by increased Syk phosphorylation, ex vivo B-cell proliferation and increased RhoA activation. Overall, our study shows for the first time that the germinal centre protein human germinal centre-associated lymphoma regulates B-cell receptor signalling in B-lymphocytes which, without appropriate control, may lead to B-cell lymphoproliferation. The human germinal centre-associated lymphoma ( HGAL) gene is expressed in germinal centre (GC) B-lymphocytes and GC-derived B-cell lymphomas [1] , [2] . In diffuse large B-cell lymphoma and classic Hodgkin lymphoma patients, HGAL expression is associated with improved survival [1] , [3] , [4] . The function of its murine homologue M17 is unknown; knockout mice demonstrated reduced-size Peyer’s patches but M17 protein was dispensable for GC formation and function [5] . In vitro studies in human lymphocytes demonstrated that HGAL decreases cell motility by interacting with F-actin, myosin II and RhoA-specific guanine nucleotide exchange factors [6] , [7] , [8] . HGAL induced RhoA effects not only on cell migration but also on gene expression [7] . These findings suggest that HGAL may contribute to the control of GC lymphocyte motility but do not explain the biological relevance of GC-specific HGAL expression. The HGAL protein harbours a modified immunoreceptor tyrosine-based activation motif (ITAM) frequently used for B-cell receptor (BCR) signal transduction. BCR signalling is initiated on antigen binding to membrane Ig, inducing receptor aggregation and Src kinase family-mediated tyrosine phosphorylation of ITAMs in signal-transducing elements Ig-α and Ig-β [9] . ITAM phosphorylation creates docking sites for Syk SH2 domains. Recruitment to the Ig-α/β facilitates Syk phosphorylation, leading to the activation of signalling molecules that couple the BCR to multiple downstream signalling pathways. Consequently, Syk has a key role in BCR signalling and its disruption leads to a block in B-cell development [10] , [11] , [12] . The presence of the ITAM, whose tyrosines can be phosphorylated by Lyn [2] , [6] , in the HGAL protein, raised a hypothesis that it might be involved in BCR signalling. We demonstrate that in vitro HGAL enhances BCR signalling by binding and increasing Syk activation. To further investigate these findings in vivo , HGAL transgenic mice were generated. Although young mice exhibited normal B-cell development, older HGAL transgenic animals progressively developed polyclonal lymphoid hyperplasia and reactive amyloid A (AA) amyloidosis. Overall, our findings implicate HGAL in regulating BCR signalling, suggesting that it may have a role in humoral immune responses. HGAL enhances intracellular BCR signalling We analysed HGAL’s effect on the BCR pathway in response to surface Ig stimulation ( Fig. 1a ). In unstimulated lymphoma cells there was no evidence for Syk, Btk and PLCγ2 phosphorylation (not shown). Following BCR stimulation, Syk, Btk and PLCγ2 phosphorylation was markedly reduced in lymphoma cell lines on knockdown of endogenous HGAL by different short interfering RNA ( Fig. 1a and Supplementary Fig. S1a ), while Ig-α/β phosphorylation was not affected (not shown). Concordantly, ectopic HGAL expression in lymphoma cells and human peripheral B-lymphocytes lacking endogenous HGAL protein resulted in increased Syk phosphorylation ( Fig. 1a ). 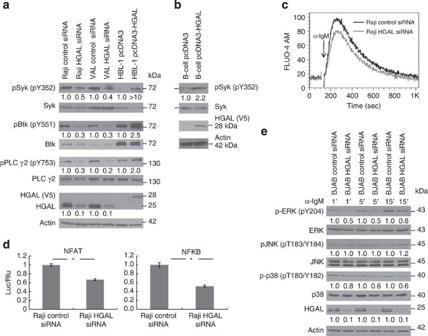Figure 1: HGAL enhances intracelular BCR signalling. Raji and VAL lymphoma cells were transfected with short interfering RNA (siRNA) for HGAL or scrambled control siRNA and HBL-1 cells (a) and normal peripheral blood B-lymphocytes (b) transfected with pcDNA3.1-HGAL or pcDNA3.1-mock plasmids for 48 h. After 1 min stimulation with goat F(ab')2 anti-human IgM, western blot of BCR receptor effectors was performed. HGAL expression and equal loading were analysed by immunoblotting with HGAL and actin antibodies. (c) Kinetic of calcium mobilization in Raji cells transfected with siRNA for HGAL or scrambled control siRNA. Arrow indicated the time point of goat F(ab')2 anti-human IgM stimulation. (d) Raji lymphoma cells were transfected with firefly luciferase reporter plasmid pNFkB-Luc or pNFAT-Luc and renilla luciferase plasmid pRL-TK and with either siRNA for HGAL or scrambled control siRNA. Forty-eight hours after transfection, the cells were stimulated for 10 min with goat F(ab')2 anti-human IgM and luciferase activities were detected with the dual luciferase assay kit. Numbers refer to luciferase activities representing three independent experiments, each performed in triplicate. * Indicate statistically significant difference (NFκBP=0.0001 and nuclear factor of activated T cellsP=0.001 by two-tailed Student’st-test). Data are presented as mean±s.d. of the mean. (e) BJAB lymphoma cells were transfected with siRNA for HGAL or scrambled control siRNA for 48 h. After stimulation with goat F(ab')2 anti-human IgM, cell lysates were used for western blot of mitogen-activated protein kinase/extracellular signal-regulated kinase pathway effectors at indicated time points. HGAL knockdown or expression and equal loading were confirmed by immunoblotting with HGAL and actin antibodies. Normalized densitometry measurements are shown below the corresponding blots. Results in (a–e) are representative of three independent experiments. NFκB, nuclear factor κB. Figure 1: HGAL enhances intracelular BCR signalling. Raji and VAL lymphoma cells were transfected with short interfering RNA (siRNA) for HGAL or scrambled control siRNA and HBL-1 cells ( a ) and normal peripheral blood B-lymphocytes ( b ) transfected with pcDNA3.1-HGAL or pcDNA3.1-mock plasmids for 48 h. After 1 min stimulation with goat F(ab')2 anti-human IgM, western blot of BCR receptor effectors was performed. HGAL expression and equal loading were analysed by immunoblotting with HGAL and actin antibodies. ( c ) Kinetic of calcium mobilization in Raji cells transfected with siRNA for HGAL or scrambled control siRNA. Arrow indicated the time point of goat F(ab')2 anti-human IgM stimulation. ( d ) Raji lymphoma cells were transfected with firefly luciferase reporter plasmid pNFkB-Luc or pNFAT-Luc and renilla luciferase plasmid pRL-TK and with either siRNA for HGAL or scrambled control siRNA. Forty-eight hours after transfection, the cells were stimulated for 10 min with goat F(ab')2 anti-human IgM and luciferase activities were detected with the dual luciferase assay kit. Numbers refer to luciferase activities representing three independent experiments, each performed in triplicate. * Indicate statistically significant difference (NFκB P =0.0001 and nuclear factor of activated T cells P =0.001 by two-tailed Student’s t -test). Data are presented as mean±s.d. of the mean. ( e ) BJAB lymphoma cells were transfected with siRNA for HGAL or scrambled control siRNA for 48 h. After stimulation with goat F(ab')2 anti-human IgM, cell lysates were used for western blot of mitogen-activated protein kinase/extracellular signal-regulated kinase pathway effectors at indicated time points. HGAL knockdown or expression and equal loading were confirmed by immunoblotting with HGAL and actin antibodies. Normalized densitometry measurements are shown below the corresponding blots. Results in ( a – e ) are representative of three independent experiments. NFκB, nuclear factor κB. Full size image In activated B-lymphocytes, Btk, PLCγ2 and BLNK constitute the calcium (Ca 2+ ) initiation complex, inducing release of intracellular Ca 2+ and activating protein kinase C, nuclear factor of activated T cells, nuclear factor κB and mitogen-activated protein kinase signalling [9] , [13] . Consequently, we examined the effects of HGAL gain and loss of function on the ability of lymphoma cells to mobilize Ca 2+ in response to BCR stimulation. Following Ig stimulation, HGAL expression in HBL-1 cells led to increased Ca 2+ mobilization (not shown), while HGAL knockdown in Raji, VAL and BJAB cells markedly reduced Ca 2+ mobilization ( Fig. 1c and Supplementary Fig. S1b ). HGAL knockdown in lymphoma cells transfected with constructs containing either nuclear factor of activated T cells or nuclear factor κB responsive luciferase reporter genes resulted in significantly decreased reporter activity ( Fig. 1d and Supplementary Fig. S1c ). HGAL knockdown in lymphoma cells also led to decreased extracellular signal-regulated kinase1/2 and p38 phosphorylation, while Jun N-terminal kinases phosphorylation was unaffected ( Fig. 1e and Supplementary Fig. S1d ), consistent with previous reports [14] . Overall, these findings show that HGAL affects BCR signalling downstream of the Ig-α/β proteins. HGAL interacts with Syk and enhances its kinase activity Syk has a major role in coupling BCR activation to downstream effectors. As Syk selectively binds to phosphorylated ITAM [10] , we examined for a potential interaction between HGAL and Syk. Endogenous Syk was detected in immunoprecipitates of endogenous HGAL from unstimulated Raji and VAL lymphoma cells ( Fig. 2a and not shown). BCR stimulation increased HGAL and Syk coimmunoprecipitation (coIP) ( Fig. 2a ). HGAL protein did not coimmunoprecipitate with Lyn, Ig-α/β p, Btk, BLNK and PLCγ2 in unstimulated and BCR-stimulated lymphoma cells (not shown). Nanoscope microscopy of unstimulated Raji cells confirmed HGAL and Syk co-localization in the cell membrane ( Fig. 2b ); BCR stimulation further increased HGAL/Syk co-localization, in concordance with the coIP findings. A glutathione S -transferase (GST) pull-down assay using purified GST-Syk, GST-Grb2 or GST and TRX-HGAL proteins demonstrated a direct, specific interaction. GST-Syk pulled-down TRX-HGAL; however, non-phosphorylated HGAL did not bind to GST-Grb2 and GST proteins ( Fig. 2c ). 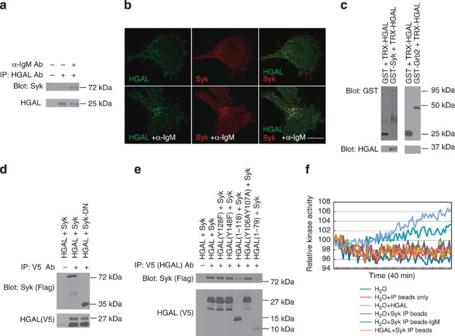Figure 2: HGAL interacts with Syk and stimulates its kinase activity. (a) Cell lysates extracted from unstimulated and goat F(ab')2 anti-human IgM stimulated (1 min) Raji lymphoma cells were subjected to immunoprecipitation with anti-HGAL or control antibodies followed by anti-HGAL and anti-Syk western blot, respectively. (b) Unstimulated or stimulated Raji cells (as described ina) were stained with HGAL (green) and Syk (red) antibodies. Scale bar, 10 μm. (c) Purified GST-Syk, GCT-Grb2 or GST proteins were incubated with TRX-HGAL protein for 12 h. The coprecipitated HGAL and Syk or Grb2 proteins were detected by western blot with anti-GST and anti-HGAL antibodies. (d) Raji cells were transfected with wild-type Syk or its dominant negative Syk-DN mutant plasmids and HGAL tagged with V5 plasmid. Cells lysates were immunoprecipitated with anti-V5 or control antibodies and analysed by western blot with anti-Syk and anti-HGAL antibodies. (e) VAL cells were transfected with Syk plasmid and V5-tagged plasmids encoding wild-type HGAL or its C-terminal truncated mutants HGAL (1–79) or HGAL(1–118), or tyrosine mutants HGAL(Y106AY107A), HGAL(Y128F) or HGAL(Y148F). Cells lysates were immunoprecipitated with anti-V5 or control antibodies and analysed by western blot with anti-Syk and anti-HGAL antibodies. (f) Syk was immunoprecipitated from unstimulated or stimulated Raji cells as described inaand used in Syk kinase activity measurement, either alone or with purified HGAL protein. Immunoprecipitates with control antibody and beads only, purified HGAL alone and water were used as negative controls. Results in (a-f) are representative of two (c) or three independent experiments. Figure 2: HGAL interacts with Syk and stimulates its kinase activity. ( a ) Cell lysates extracted from unstimulated and goat F(ab')2 anti-human IgM stimulated (1 min) Raji lymphoma cells were subjected to immunoprecipitation with anti-HGAL or control antibodies followed by anti-HGAL and anti-Syk western blot, respectively. ( b ) Unstimulated or stimulated Raji cells (as described in a ) were stained with HGAL (green) and Syk (red) antibodies. Scale bar, 10 μm. ( c ) Purified GST-Syk, GCT-Grb2 or GST proteins were incubated with TRX-HGAL protein for 12 h. The coprecipitated HGAL and Syk or Grb2 proteins were detected by western blot with anti-GST and anti-HGAL antibodies. ( d ) Raji cells were transfected with wild-type Syk or its dominant negative Syk-DN mutant plasmids and HGAL tagged with V5 plasmid. Cells lysates were immunoprecipitated with anti-V5 or control antibodies and analysed by western blot with anti-Syk and anti-HGAL antibodies. ( e ) VAL cells were transfected with Syk plasmid and V5-tagged plasmids encoding wild-type HGAL or its C-terminal truncated mutants HGAL (1–79) or HGAL(1–118), or tyrosine mutants HGAL(Y106AY107A), HGAL(Y128F) or HGAL(Y148F). Cells lysates were immunoprecipitated with anti-V5 or control antibodies and analysed by western blot with anti-Syk and anti-HGAL antibodies. ( f ) Syk was immunoprecipitated from unstimulated or stimulated Raji cells as described in a and used in Syk kinase activity measurement, either alone or with purified HGAL protein. Immunoprecipitates with control antibody and beads only, purified HGAL alone and water were used as negative controls. Results in ( a - f ) are representative of two ( c ) or three independent experiments. Full size image To determine whether the Syk tandem SH2 domains mediate interaction with HGAL protein, we transiently co-transfected wild-type HGAL with truncated Syk encoding the tandem SH2 domains (amino acids 1–261) into Raji and 293T cells and repeated the coIP experiments. Truncated Syk protein was detected in the HGAL immunoprecipitates ( Fig. 2d and Supplementary Fig. S2a ), indicating that HGAL protein interacts with the Syk tandem SH2 domains. To determine the HGAL interacting domain, HGAL mutants encoding N-terminal 79 (1–79) or 118 (1–118) aa segments and tyrosine mutants (Y128F, Y148F and Y106AY107A) ( Supplementary Fig. S2b ) were co-transfected with the wild-type Syk into VAL and 293T cells and coIP experiments were repeated ( Fig. 2e and Supplementary Fig. S2c ). Individual mutations of HGAL tyrosines and HGAL truncations did not affect Syk binding, suggesting that the first 79aa of HGAL were sufficient to mediate Syk binding. We next examined whether the HGAL protein stimulates Syk kinase activity. Syk protein was immunoprecipitated from BCR-stimulated or unstimulated Raji cells and used in the kinase assay, either alone or with purified HGAL protein ( Fig. 2f ). No Syk kinase activity was observed in unstimulated cells, even in the presence of HGAL protein. In stimulated cells, addition of HGAL protein markedly increased Syk kinase activity, suggesting that HGAL binding to Syk enhances its kinase activity in BCR-stimulated cells, underlying the observed increased Syk autophosphorylation and activation of its downstream effectors. HGAL gain-of-function mouse model To examine HGAL effects on the immune system and BCR signalling in vivo , a Sca1-HGAL plasmid encoding human HGAL complementary DNA (cDNA) under the control of the mouse Ly-6E.1 promoter [15] ( Fig. 3a ) was used to generate a transgenic mouse model in which HGAL is expressed in Sca1 + haematopoietic stem (HSC)/progenitor cells and Sca1 + fraction of mature B cells of C57BL/6xCBA mice [16] . A similar approach recapitulated gene functions and generated animal models highly similar to human diseases [17] , [18] , [19] . Two independent Sca1-HGAL founder lines (102A and 102B) exhibited normal embryonic and postnatal development and were used to characterize the transgenic mice phenotype. 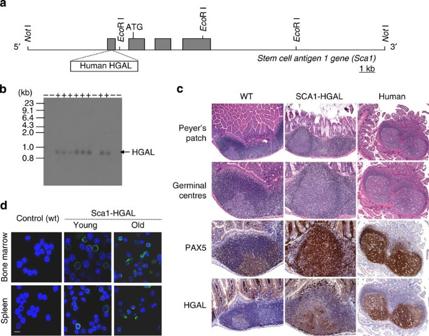Figure 3: HGAL gain-of-function mouse model. (a) Schematic representation of the genomic structure of the mouseSca1locus and the Sca1-HGAL transgenic vector used to generate transgenic animals. (b) Identification of the transgenic mice (n=75) by Southern analysis of tail snip DNA afterEcoRI digestion. Sca1-HGAL is indicated. (c) HGAL expression in Sca1-HGAL mice. BM and spleen cells of control (n=3) and Sca1-HGAL mice (n=3) were stained with anti-V5 antibody (green) and 4',6-diamidino-2-phenylindole (blue) and examined under a microscope. Data are representative of three independent experiments. Scale bar, 10 μm (d). Representative sections of ileum show increased-sized Peyer’s patches and prominent GCs stained with PAX5 and HGAL in Sca1-HGAL compared with control mice. All mouse images were photographed at comparable magnifications: X100, Peyer’s patches panels; X300, remaining panels. Human Peyer’s patches are shown for comparison (X40, Peyer’s patches panel, X80, remaining panels). Figure 3: HGAL gain-of-function mouse model. ( a ) Schematic representation of the genomic structure of the mouse Sca1 locus and the Sca1-HGAL transgenic vector used to generate transgenic animals. ( b ) Identification of the transgenic mice ( n =75) by Southern analysis of tail snip DNA after Eco RI digestion. Sca1-HGAL is indicated. ( c ) HGAL expression in Sca1-HGAL mice. BM and spleen cells of control ( n =3) and Sca1-HGAL mice ( n =3) were stained with anti-V5 antibody (green) and 4',6-diamidino-2-phenylindole (blue) and examined under a microscope. Data are representative of three independent experiments. Scale bar, 10 μm ( d ). Representative sections of ileum show increased-sized Peyer’s patches and prominent GCs stained with PAX5 and HGAL in Sca1-HGAL compared with control mice. All mouse images were photographed at comparable magnifications: X100, Peyer’s patches panels; X300, remaining panels. Human Peyer’s patches are shown for comparison (X40, Peyer’s patches panel, X80, remaining panels). Full size image A Southern blot comparison of the endogenous M17 and transgenic human HGAL hybridization signals indicated transgene copy numbers ranging from 2 to 4 ( Fig. 3b ). Flow cytometry studies revealed that only a fraction of B220 splenocytes expressed Sca1. Similar fractions of B220 splenocytes in young Sca1-HGAL (4- to 8-week-old) and control mice expressed Sca1 ( Supplementary Fig. S3a ). While there was a tendency for a smaller Sca1 expressing fraction of B220 splenocytes in older (starting at 12 months of age) Sca1-HGAL mice compared with control animals, it was not statistically significant ( Supplementary Fig. S3a ). Immunofluorescence studies using antibody to the V5 tag, fused to HGAL in the plasmid used to generate the transgenic animal, detected ectopically expressed human HGAL in both bone marrow (BM) and spleen cells ( Fig. 3c ), with no difference in expression between young and old animals. HGAL expression was not detected in either mature myeloid, monocyte and T-cell lineages or in the wild-type controls. Overall, HGAL protein expression levels were similar to levels observed in the human U2OS cell line transfected with the same HGAL plasmid used to generate the transgenic construct ( Supplementary Fig. S3b ). There was no difference in the endogenous M17 messenger RNA (mRNA) expression between Sca1-HGAL and littermate splenocytes ( Supplementary Fig. S3c ). Lymphoid hyperplasia and amyloidosis in Sca1-HGAL mice A total of 75 transgenic animals were analysed. Compared with age-matched controls, 8-week-old Sca1-HGAL animals did not show any visible changes within the major haematopoietic compartments (BM, spleen, thymus, peripheral blood and lymph nodes (LNs)) by flow cytometry and histological examinations ( Fig. 4a , Supplementary Fig. S4 ). Immunization with sheep red blood cells led to GC formation in both transgenic and wild-type mice. Flow cytometry analyses did not reveal statistically significant differences in the number of splenic B220 + PNA + Fas + GL7 + GC B cells between the Sca1-HGAL and control animals ( Supplementary Fig. S5a ). Immunohistochemistry also did not reveal differences in the size and number of GCs in the spleens of immunized Sca1-HGAL and control mice ( Supplementary Fig. S5b ), indicating that young Sca1-HGAL mice respond normally to T-cell-dependent antigen stimulation. 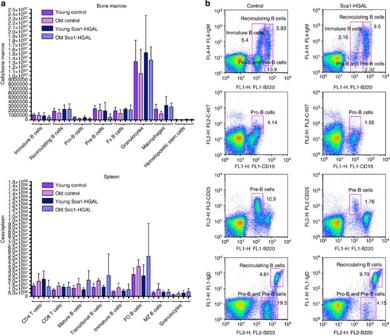Figure 4: Analysis of the BM and spleen cell lineages in the Sca1-HGAL mice. Cells from the BM and spleen of young (8 weeks) and old (more than 7-month-old) age-matched Sca1-HGAL mice and wild-type controls (n=11 in each group) were analysed by flow cytometry. (a) Total cell number of the indicated cell sub-populations in the BM and spleens of the young and old Sca1-HGAL and control mice. Data are presented as mean±s.d. of the mean. (b) Representative FACS plots of 12-month-old Sca1-HGAL mice are displayed. FACS definition of B-cell developmental stages was performed according to Kwonet al.37 Figure 4: Analysis of the BM and spleen cell lineages in the Sca1-HGAL mice. Cells from the BM and spleen of young (8 weeks) and old (more than 7-month-old) age-matched Sca1-HGAL mice and wild-type controls ( n =11 in each group) were analysed by flow cytometry. ( a ) Total cell number of the indicated cell sub-populations in the BM and spleens of the young and old Sca1-HGAL and control mice. Data are presented as mean±s.d. of the mean. ( b ) Representative FACS plots of 12-month-old Sca1-HGAL mice are displayed. FACS definition of B-cell developmental stages was performed according to Kwon et al . [37] Full size image Starting at 12 months of age, the Sca1-HGAL mice demonstrated increased-sized Peyer’s patches compared with control animals ( Fig. 3d ) and expressed HGAL protein at levels similar to ones observed in human Payer’s patches. These animals also exhibited non-statistically significant decrease in number of BM immature and pro- and pre-B-cells at the expense of recirculating B cells (B220 + IgD hi ) ( Fig. 4a ). All the Sca1-HGAL mice became ill, showing decreased spontaneous movements in the cage, increased respiratory rates, piloerection and shivering, and died between 12 and 22 months, exhibiting statistically significant shorter overall survival ( Fig. 5a ). 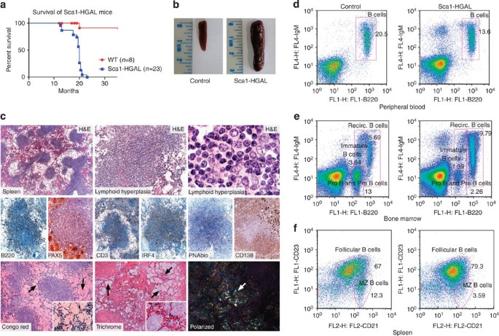Figure 5: B-cell lymphoid hyperplasia in Sca1-HGAL mice. (a) Kaplan–Meier overall survival plots of Sca1-HGAL mice. The total numbers of mice analysed in each group were eight wild-type control mice and 23 Sca1-HGAL transgenic mice. Differential survival in Sca1-HGAL and control mice was analysed using the log-rank test (P=0.0000003). (b) Sca1-HGAL mice develop massive splenomegaly. Data is representative of pathologic analysis of 36 Sca1-HGAL transgenic mice. (c) Representative sections of spleen of Sca1-HGAL mice show overall preservation of microscopic architecture; however, the splenic sinusoids were dilated and distorted by large quantities of proteinaceous deposits (spleen haematoxylin and eosin (H&E) panel original magnification I X40; lymphoid hyperplasia panels original magnifications X100 and X400). These deposits were found adjacent to lymphoid hyperplasia, which was highlighted by B220 (weak positive staining) and PAX5 representing B cells, and a smaller proportion of CD3-positive T-cells. Staining for IRF4 highlighted T-cell areas in addition to a few scattered plasmacytoid cells while PNAbio (a GC marker) showed no significant staining to indicate GC formation. CD138 showed weak expression in the B cells without the intense expression typically seen in plasma cells (B220, PAX5, CD3, IRF4, PNAbio and CD138 panels, X200 original magnification). Congo red (orange staining) and trichrome (greyish-blue) stains highlight amyloid deposits, which under polarized light, showed the characteristic apple-green birefringence (X400 original magnification). (d-f) Representative FACS plots of peripheral blood (d), BM (e) and spleen (f) lymphocytes from Sca1-HGAL mice with lymphoid hyperplasia (n=15) and control littermates (n=15). Figure 5: B-cell lymphoid hyperplasia in Sca1-HGAL mice. ( a ) Kaplan–Meier overall survival plots of Sca1-HGAL mice. The total numbers of mice analysed in each group were eight wild-type control mice and 23 Sca1-HGAL transgenic mice. Differential survival in Sca1-HGAL and control mice was analysed using the log-rank test ( P =0.0000003). ( b ) Sca1-HGAL mice develop massive splenomegaly. Data is representative of pathologic analysis of 36 Sca1-HGAL transgenic mice. ( c ) Representative sections of spleen of Sca1-HGAL mice show overall preservation of microscopic architecture; however, the splenic sinusoids were dilated and distorted by large quantities of proteinaceous deposits (spleen haematoxylin and eosin (H&E) panel original magnification I X40; lymphoid hyperplasia panels original magnifications X100 and X400). These deposits were found adjacent to lymphoid hyperplasia, which was highlighted by B220 (weak positive staining) and PAX5 representing B cells, and a smaller proportion of CD3-positive T-cells. Staining for IRF4 highlighted T-cell areas in addition to a few scattered plasmacytoid cells while PNAbio (a GC marker) showed no significant staining to indicate GC formation. CD138 showed weak expression in the B cells without the intense expression typically seen in plasma cells (B220, PAX5, CD3, IRF4, PNAbio and CD138 panels, X200 original magnification). Congo red (orange staining) and trichrome (greyish-blue) stains highlight amyloid deposits, which under polarized light, showed the characteristic apple-green birefringence (X400 original magnification). ( d - f ) Representative FACS plots of peripheral blood ( d ), BM ( e ) and spleen ( f ) lymphocytes from Sca1-HGAL mice with lymphoid hyperplasia ( n =15) and control littermates ( n =15). Full size image Macroscopic analysis of these animals revealed massive splenomegaly ( Fig. 5b ). The overall microscopic architecture of the spleen was preserved; however, the splenic sinusoids were dilated and distorted by large quantities of proteinaceous deposits, which were also present surrounding small and medium-calibre splenic blood vessels ( Fig. 5c ). These deposits were found adjacent to expanded white-pulp areas showing lymphoid hyperplasia with preserved periarteriolar lymphoid sheaths. Immunohistochemistry using B220 and PAX5 antibodies highlighted a significant proportion of the expanded white pulp representing B cells, whereas CD3 highlighted a slightly smaller proportion of T cells. B220 staining was weak compared with that of PAX5, although both stains showed an equivalent distribution of B cells. Staining for IRF4 highlighted T-cell areas in addition to a few scattered plasmacytoid cells. PNAbio showed no significant staining within the white-pulp, suggesting that white-pulp expansions represented lymphoid hyperplasia without GC formation ( Fig. 5c ). Control animals showed a similar distribution of B and T cells within the white-pulp, although without lymphoid hyperplasia ( Supplementary Fig. S6a ). In both Sca1-HGAL and control animals, CD38 (not shown) and CD138 showed weak expression in the B cells without the intense expression typically seen in plasma cells ( Fig. 5c and Supplementary Fig. S6a ). Flow cytometry also did not demonstrate differences in the number and percentage of B220 lo CD138+ splenic cells between young and old Sca1-HGAL and control mice ( Supplementary Fig. S6b ). In contrast, flow cytometry analysis detected IgM+ B-cells in peripheral blood and BM ( Fig. 5d ), confirming that the observed splenic lymphoid hyperplasia was due to follicular (FO) B cells ( Fig. 5f ). The percentage of Sca1 + Lin − cells in BM did not increase in Sca1-HGAL mice compared with normal littermates (data not shown). Analysis of the B-1 lymphocyte population in the older animals revealed a significant decrease in B-1 cell number and percentage in the spleen and a significant increase in the LN of the Sca1-HGAL mice compared with normal littermates ( Supplementary Fig. S4 ). There was no difference in the number and percentage of B-1 and B-1a cells in the BM and peritoneum between the Sca1-HGAL and control animals. Congo red and trichrome stains of the spleens for amyloid showed distinctive positive staining of the proteinaceous deposits; Congo red showed the characteristic muted orange colour on light microscopy and exhibited apple-green birefringence under polarized light. Similarly, the trichrome stain showed a greyish-blue colour, consistent with amyloid deposition and in contrast to the bright turquoise blue that is typically demonstrated by collagen ( Fig. 5c ). Tissue sections from multiple organs including the kidney, liver, lung and small intestine showed similar massive amyloid deposition ( Supplementary Fig. S7a,b ). Sections of the kidney, liver and lung showed preservation of the normal architecture with modest mixed lymphoid infiltrates that were absent in control animals. Massive amyloid deposition was observed in all renal glomeruli, as well as the interstitium. Amyloid deposition was also seen surrounding small and medium calibre blood vessels in the kidneys, lung and liver, but not the heart. Electron microscopy of spleen specimens confirmed the presence of amyloid deposits ( Supplementary Fig. S7c,d ). Liquid chromatography tandem mass spectrometry analysis of the kidney and spleen specimens showed that the most abundant pathogenic protein in the amyloid deposits was serum amyloid-associated protein-2, consistent with AA amyloidosis ( Fig. 6 ). Analysis of serum amyloid-associated protein-2 peptide sequences revealed the absence of 33 aa of the C terminus, suggesting these residues were cleaved during the amyloidogenesis, similar to what has been described in human AA amyloidosis [20] . Like in human amyloidosis, constituents of many human amyloid types (apolipoprotein E, apolipoprotein A-IV, serum amyloid P-component and apolipoprotein A-I) were also detected in the amyloid deposits in the Sca1-HGAL mice. 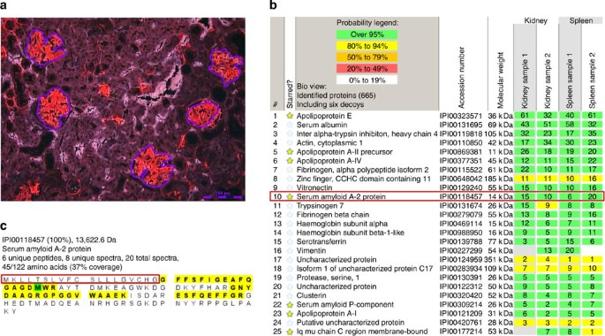Figure 6: Analysis of amyloid fibrils. (a) Congo red-stained kidney specimen viewed under fluorescent light source with bright red areas representing amyloid deposits. Purple coloured lines-areas microdissected for MS-based proteomic analysis. (b) Results of MS-based proteomic analysis of amyloid plaques from the kidney and spleen specimens in two independent microdissections. The identified proteins are listed according to their relative abundance, with top 25 from a total of 720 proteins shown. The columns show the protein name, the UnitProt identifier (protein accession number in the UniProt database,http://www.uniprot.org/), the molecular weight of the protein, two microdissections of the kidney specimen and two microdissections of the spleen specimen. The numbers indicate number of total peptide spectra identified for each protein. The amyloid-associated proteins are identified by yellow stars. The peptides representing the serum amyloid A-2 protein (red box) are the primary cause of amyloid deposits in the Sca1-HGAL mouse model. (c) serum amyloid-associated protein-2 (SAA2) protein coverage in the Sca1-HGAL mouse amyloidosis model. The amino-acid (aa) sequence of the SAA2_MOUSE is provided. The yellow highlights indicate the parts of the protein that were identified by the liquid chromatography tandem mass spectrometry. The first 19 aa represent the N terminus signal peptide of the SAA2_MOUSE (red box) cleaved before the mature SAA2_MOUSE is secreted into the circulation, and thus is not expected to be part of the amyloid deposits. The peptides missing in the middle of the protein are unlikely to be detected by liquid chromatography tandem mass spectrometry due to abundance of numerous trypsin cutting sites. Figure 6: Analysis of amyloid fibrils. ( a ) Congo red-stained kidney specimen viewed under fluorescent light source with bright red areas representing amyloid deposits. Purple coloured lines-areas microdissected for MS-based proteomic analysis. ( b ) Results of MS-based proteomic analysis of amyloid plaques from the kidney and spleen specimens in two independent microdissections. The identified proteins are listed according to their relative abundance, with top 25 from a total of 720 proteins shown. The columns show the protein name, the UnitProt identifier (protein accession number in the UniProt database, http://www.uniprot.org/ ), the molecular weight of the protein, two microdissections of the kidney specimen and two microdissections of the spleen specimen. The numbers indicate number of total peptide spectra identified for each protein. The amyloid-associated proteins are identified by yellow stars. The peptides representing the serum amyloid A-2 protein (red box) are the primary cause of amyloid deposits in the Sca1-HGAL mouse model. ( c ) serum amyloid-associated protein-2 (SAA2) protein coverage in the Sca1-HGAL mouse amyloidosis model. The amino-acid (aa) sequence of the SAA2_MOUSE is provided. The yellow highlights indicate the parts of the protein that were identified by the liquid chromatography tandem mass spectrometry. The first 19 aa represent the N terminus signal peptide of the SAA2_MOUSE (red box) cleaved before the mature SAA2_MOUSE is secreted into the circulation, and thus is not expected to be part of the amyloid deposits. The peptides missing in the middle of the protein are unlikely to be detected by liquid chromatography tandem mass spectrometry due to abundance of numerous trypsin cutting sites. Full size image To examine whether the observed lymphoid hyperplasia were of clonal origin, DNA extracted from the splenic B-lymphocytes from Sca1-HGAL mice were subjected to Southern blot using the 3′ J H 4 probe. No Ig heavy chain (IgH) gene rearrangements were detected ( Supplementary Fig. S8a ). Polymerase chain reactions followed by direct sequencing or cloning and sequencing of multiple molecular clones also failed to detect predominant monoclonal products ( Supplementary Fig. S8b ), further indicating that the observed lymphoid hyperplasia were of polyclonal origin. Cytogenetic and fluorescence in situ hybridization studies of the splenic B-lymphocytes from lymphoid hyperplasia demonstrated normal karyotypes without evidence for Bcl2-IgH translocation (not shown). Sca1-HGAL mice display hypergammaglobulinemia The presence of polyclonal FO B-cell lymphoid hyperplasia in the Sca1-HGAL transgenic mice pointed to possible immune stimulation, potentially leading to hypergammaglobulinemia. The non-immunized Sca1-HGAL mice produced antibodies of all isotypes and IgG titres tended to be higher than in the wild-type controls, reaching statistical difference for IgG1 isotype ( Fig. 7a ). 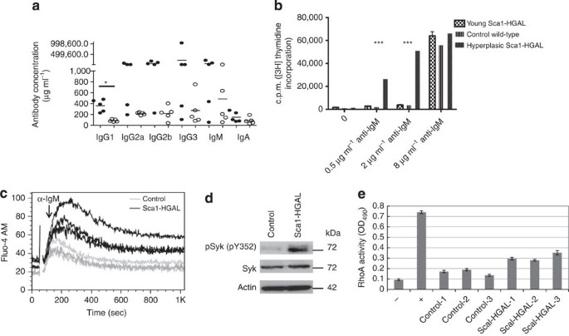Figure 7: Hypergammaglobulinemia and enhanced BCR and RhoA signalling in the Sca1-HGAL mice. (a) Ig isotype titres in the serum of 14-month-old unimmunized control (open circles) and Sca1-HGAL (black circles) mice analysed by enzyme-linked immunosorbent assay.n=5 per group. * IndicatesP=0.0007 by two-tailed Student’st-test. (b)Ex vivoB-cell proliferation in response to surface Ig stimulation. Purified splenic B cells from wild-type mice, young Sca1-HGAL transgenic mice without lymphoid hyperplasia and Sca1-HGAL transgenic mice with lymphoid hyperplasia (three animals in each group) were stimulated with the indicated concentrations of an anti-IgM antibody and cell proliferation assessed by [3H]thymidine incorporation in triplicates. Shown is mean±s.e.m. *** Indicates statistically significant difference: for 0.5 μg ml−1anti-IgMP=0.000004 and for 2 μg ml−1anti-IgMP=0.00000007 by two-way analysis of variance test. (c) Kinetic of calcium mobilization measured by flow cytometry in purified spleen B-lymphocytes from three Sca1-HGAL transgenic mice with lymphoid hyperplasia (black) and three wild-type control mice (grey). Arrow indicates the time point of stimulation with goat F(ab')2 anti-mouse IgM. (d) Purified spleen B-lymphocytes from Sca1-HGAL transgenic or control mice stimulated with goat F(ab')2 anti-mouse IgM for 1 min were used for western blot with pSyk (pY352) and total Syk antibodies. Equal loading was confirmed by immunoblotting with actin antibodies. (e) Purified spleen B cells from Sca1-HGAL transgenic or wild-type control mice stimulated with 1 μg ml−1lysophosphatidic acid for 45 seconds were used for RhoA activity measurement in triplicates; lysis buffer served as negative control and RhoA protein as a positive control. Shown is mean±s.d. Results indandeare representative of three independent experiments. Figure 7: Hypergammaglobulinemia and enhanced BCR and RhoA signalling in the Sca1-HGAL mice. ( a ) Ig isotype titres in the serum of 14-month-old unimmunized control (open circles) and Sca1-HGAL (black circles) mice analysed by enzyme-linked immunosorbent assay. n =5 per group. * Indicates P =0.0007 by two-tailed Student’s t -test. ( b ) Ex vivo B-cell proliferation in response to surface Ig stimulation. Purified splenic B cells from wild-type mice, young Sca1-HGAL transgenic mice without lymphoid hyperplasia and Sca1-HGAL transgenic mice with lymphoid hyperplasia (three animals in each group) were stimulated with the indicated concentrations of an anti-IgM antibody and cell proliferation assessed by [ 3 H]thymidine incorporation in triplicates. Shown is mean±s.e.m. *** Indicates statistically significant difference: for 0.5 μg ml −1 anti-IgM P =0.000004 and for 2 μg ml −1 anti-IgM P =0.00000007 by two-way analysis of variance test. ( c ) Kinetic of calcium mobilization measured by flow cytometry in purified spleen B-lymphocytes from three Sca1-HGAL transgenic mice with lymphoid hyperplasia (black) and three wild-type control mice (grey). Arrow indicates the time point of stimulation with goat F(ab')2 anti-mouse IgM. ( d ) Purified spleen B-lymphocytes from Sca1-HGAL transgenic or control mice stimulated with goat F(ab')2 anti-mouse IgM for 1 min were used for western blot with pSyk (pY352) and total Syk antibodies. Equal loading was confirmed by immunoblotting with actin antibodies. ( e ) Purified spleen B cells from Sca1-HGAL transgenic or wild-type control mice stimulated with 1 μg ml −1 lysophosphatidic acid for 45 seconds were used for RhoA activity measurement in triplicates; lysis buffer served as negative control and RhoA protein as a positive control. Shown is mean±s.d. Results in d and e are representative of three independent experiments. Full size image Enhanced BCR signalling in lymphoid hyperplasia splenocytes The observed lymphoid hyperplasia in the Sca1-HGAL mice might be attributed to increased B-cell proliferation due to enhanced BCR signalling or to promotion of B-cell survival. To differentiate between these mechanisms, we examined ex vivo B-cell proliferation in response to BCR stimulation ( Fig. 7b ). There was no difference in cell proliferation rates between control and young Sca1-HGAL mouse groups at all analysed IgM concentrations. In contrast, B-cells from Sca1-HGAL mice with lymphoid hyperplasia demonstrated increased proliferation to 0.5 and 2 μg ml −1 anti-IgM antibody concentrations compared with both wild-type controls and young transgenic mice. However, B-cell proliferation was similar in all the three types of animals at saturating 8 μg ml −1 anti-IgM antibody concentrations. Splenic B-cell surface Ig expression was similar in all the three types of analysed animals (not shown). These findings suggest that B-lymphocytes from Sca1-HGAL mice with lymphoid hyperplasia show enhanced sensitivity to surface Ig stimulation. Concordantly, increased Ca 2+ mobilization ( Fig. 7c ) and Syk phosphorylation ( Fig. 7d ) were observed in the BCR-stimulated B-cells from Sca1-HGAL mice with lymphoid hyperplasia compared with control animals. In contrast, isolated B220+ splenocytes from Sca1-HGAL transgenic and control mice supplemented only with 5% FCS exhibited a similar in vitro overtime death rate ( Supplementary Fig. S9 ), suggesting that HGAL does not promote B-cell survival in the Sca1-HGAL mice. RhoA activation in Sca1-HGAL transgenic mice Our previous in vitro studies demonstrated that HGAL induces RhoA activation in human B-cells [7] . Consequently, we examined the levels of GTP-bound RhoA in B-cell splenocytes isolated from Sca1-HGAL transgenic mice with and without lymphoid hyperplasia. RhoA-GTP levels were significantly higher in Sca1-HGAL B-cells from spleens with versus without lymphoid hyperplasia ( P =0.006, analysed by two-tailed Student’s t -test) ( Fig. 7e ), corroborating the observed activation of this pathway in human B cells. Transcriptome changes in Sca1-HGAL transgenic mice To comprehensively assess the global effect of HGAL on lymphocyte functions and the observed lymphoproliferation, we performed gene expression profiling using isolated CD22+B220+ splenocytes from adult Sca1-HGAL mice with hyperplastic follicles and wild-type littermates (four samples each). In supervised analyses using significance analysis of microarrays [21] at a 10% false discovery rate (FDR), we identified 981 genes with significantly increased expression in B-splenocytes from adult Sca1-HGAL mice with lymphoid hyperplasia compared with controls ( Supplementary Data 1 ). Fig. 8a depicts 107 of these genes ( Supplementary Data 2 ), focusing on those with at least threefold change between the specimens from Sca1-HGAL transgenic and control mice. In concordance with HGAL’s role in regulating lymphocyte motility, gene expression profiles in the Sca1-HGAL mice with lymphoid hyperplasia apparently reflect ‘Cell Movement’ ( P =5.46e-9, IPA) and ‘Migration of Cells’ ( P =0.0001, IPA) as evidenced by significant overlap with the corresponding pathways using the Ingenuity Pathway Analysis knowledge base. Sca1-HGAL B-splenocytes also exhibited decreased mRNA expression of regulator of G-protein signalling 13 and 18 (RGS13 and RGS18), whose downregulation may enhance the signalling activity of G-proteins potentially enhancing RhoA activation. 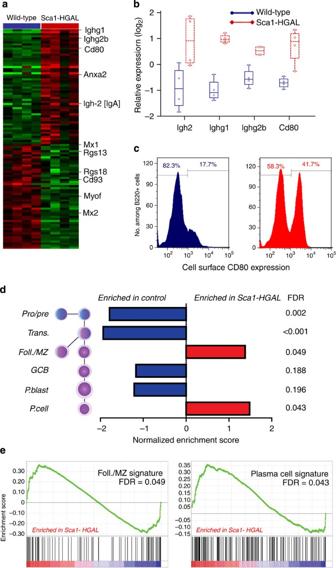Figure 8: Transcriptional signatures evokedin vivowithin B-cell lymphoid hyperplasia in the Sca1-HGAL mice. (a) Genes significantly induced or repressed within purified B220+ splenocytes of Sca1-HGAL mice in comparison with wild-type littermates, as determined by significance analysis of microarrays using an FDR 10% and demonstrating at least threefold change. Each row represents a separate gene and each column a separate mRNA sample from each of eight mice, with four mice from within each group. The level of expression of each gene in each sample, relative to the mean level of expression of that gene across all the samples, is represented using a red–green colour scale, extending from fluorescence ratios of 0.25 to 4 (−2 to +2 in log base 2 units). Selected genes are highlighted. (b) Depicted are the relative mRNA expression levels for selected genes exhibiting significant differential expression froma, includingIgh-2(IgA),Ighg1(IgG1),Ighg2b(IgG2b) andCd80(CD80). These genes were independently assessed for differential expression of the corresponding proteins (in parentheses), as depicted inFig. 7a, and panelc. (c) Induction of CD80 cell surface protein expression in B-cell splenocytes of the Sca1-HGAL mice measured by flow cytometry. Data are representative of three mice. (d) GSEA of the relative representation of differentiation states within Sca1-HGAL compared with control B-cells. Gene expression data from Sca1-HGAL B cells showed significant enrichment for signatures corresponding to both FO/MZ and plasma cell normal murine B-cell differentiation states, suggesting an over-representation of these states within Sca1-HGAL cells. Signatures corresponding to other differentiation states were significantly enriched in control B cells, suggesting a relative under-representation in Sca1-HGAL B cells. (e) Detailed view of GSEA results, showing a strong bias of genes from normal FO/MZ B cells (left panel) and plasma cells (right panel) in Sca1-HGAL B cells compared with control B cells. Figure 8: Transcriptional signatures evoked in vivo within B-cell lymphoid hyperplasia in the Sca1-HGAL mice. ( a ) Genes significantly induced or repressed within purified B220+ splenocytes of Sca1-HGAL mice in comparison with wild-type littermates, as determined by significance analysis of microarrays using an FDR 10% and demonstrating at least threefold change. Each row represents a separate gene and each column a separate mRNA sample from each of eight mice, with four mice from within each group. The level of expression of each gene in each sample, relative to the mean level of expression of that gene across all the samples, is represented using a red–green colour scale, extending from fluorescence ratios of 0.25 to 4 (−2 to +2 in log base 2 units). Selected genes are highlighted. ( b ) Depicted are the relative mRNA expression levels for selected genes exhibiting significant differential expression from a , including Igh-2 (IgA), Ighg1 (IgG1), Ighg2b (IgG2b) and Cd80 (CD80). These genes were independently assessed for differential expression of the corresponding proteins (in parentheses), as depicted in Fig. 7a , and panel c . ( c ) Induction of CD80 cell surface protein expression in B-cell splenocytes of the Sca1-HGAL mice measured by flow cytometry. Data are representative of three mice. ( d ) GSEA of the relative representation of differentiation states within Sca1-HGAL compared with control B-cells. Gene expression data from Sca1-HGAL B cells showed significant enrichment for signatures corresponding to both FO/MZ and plasma cell normal murine B-cell differentiation states, suggesting an over-representation of these states within Sca1-HGAL cells. Signatures corresponding to other differentiation states were significantly enriched in control B cells, suggesting a relative under-representation in Sca1-HGAL B cells. ( e ) Detailed view of GSEA results, showing a strong bias of genes from normal FO/MZ B cells (left panel) and plasma cells (right panel) in Sca1-HGAL B cells compared with control B cells. Full size image We also observed significant induction of BCR pathway components in the Sca1-HGAL mice ( Fig. 8a ), including Ig heavy chain genes (Ighg1, Igh-2 (IgA), Ighg2b, Ighg2c), corroborating our observation of serum hypergammaglobulinemia ( Fig. 7a ). Within these lymphoid hyperplasias we also observed significant induction of CD80 ( Fig. 8b ), which costimulates T-lymphocytes, a finding which we confirmed at the protein level ( Fig. 8c ), demonstrating CD80 expression in a fraction of B-lymphocytes. No significant differences in expression levels of mRNAs for CD86 (B7-2), CD69, CD5 or MHC-II antigens were detected. To evaluate the relative representation of normal differentiation states within splenocytes from Sca1-HGAL mice with hyperplastic follicles compared with B cells from wild-type littermates, we utilized gene set enrichment analysis (GSEA) of transcriptional profiling data. Classification signatures from normal murine stages of B-cell differentiation were obtained from Green et al . [22] to assess expression bias in Sca1-HGAL compared with control B cells. Gene expression signature corresponding to both the normal FO/marginal zone (FO/MZ) and the plasma cell B-cell differentiation states were significantly enriched in Sca1-HGAL B-cells ( Fig. 8d ). Conversely, signatures corresponding to the remaining differentiation states were significantly enriched in control B cells, suggesting a relative over-representation of B cells at the FO/MZ and plasma cell differentiation states in Sca1-HGAL mice with hyperplastic follicles. To further validate the role of HGAL in these B-cell differentiation states, we performed a reciprocal analysis of Sca1-HGAL signatures in transcriptional profiling data from normal murine B cells [22] . Genes found to be highly expressed in Sca1-HGAL B cells compared with control B cells ( Fig. 8a ) were tested for enrichment in normal FO/MZ and plasma B cells and compared with B cells of other differentiation states. This revealed a significant enrichment of HGAL-induced genes in normal FO/MZ B cells, but not in normal plasma cells, compared with other differentiation states ( Supplementary Fig. S10a–c ). The lack of significant enrichment in normal plasma cells is likely the result of downregulation of a subset of HGAL-induced genes within this differentiation state. Together, these results suggest that Sca1-HGAL B cells possess transcriptional signatures indicative of an over-representation of FO/MZ B cells and plasma cells. However, immunohistochemistry and flow cytometry studies did not show an increase in plasma cells in the lymphoid hyperplasia observed in the Sca1-HGAL mice, suggesting that the B220+ cells may be poised towards plasma cell differentiation; however, induced transcriptional changes characteristic to plasma cells were insufficient to lead to plasma cell differentiation. Indeed, the observed transcriptional signatures lacked expression of PRDM1 and XBP1 , genes necessary for plasma cell genesis. Furthermore, normal murine FO/MZ B cells had significantly enriched expression of HGAL-induced genes, suggesting that HGAL may have a role in normal FO/MZ B-cell biology. We also compared the transcriptional responses evoked by HGAL in B-cell lymphoid hyperplasia of Sca1-HGAL mice to those induced in other B-cell tumours at various stages of the B-cell lineage, with a focus on those arrested at the GC and beyond [23] , [24] . Notably, genes induced in the lymphoid hyperplasia in the Sca1-HGAL mice significantly overlapped those upregulated in murine GC-derived lymphomas driven by Bcl6 (ref. 24 ) ( P =2.48e−4 by hypergeometric test) ( Supplementary Fig. S10d ) and were also enriched for those uniformly repressed within plasma cell tumours driven by Myc/Bcl-xL [23] ( P =1.8e−12 by hypergeometric test) ( Supplementary Fig. S10e ), suggesting a distinct regulatory programme in these hyperplasia leading to Ig secretion. The outcome of BCR stimulation is diverse and is determined by the maturation state of the cell, the nature and quantity of the antigen, signals from coreceptors and the magnitude and duration of BCR signalling. An ‘on-off’ mode of BCR signal transduction would not allow for diverse cellular responses. Fine-tuning the magnitude and duration of BCR signalling and preferential activation of specific downstream signalling components by adaptor proteins selectively expressed during B-cell development is of paramount importance for B-cell functional plasticity [25] , [26] . We demonstrate that the GC-specific adaptor HGAL regulates BCR signalling by direct binding and activation of Syk. While HGAL is not necessary for GC formation [5] , HGAL transgenic animals exhibited increased-size Peyer’s patches, a finding corroborating the reduced-size Peyer’s patches in the M17 knockout mice [5] . This observation suggests a specific function of HGAL in Peyer’s patches. Furthermore, it is possible that the increased-size HGAL expressing Peyer‘s patches may contribute to systemic lymphoid hyperplasia and subsequent development of AA amyloidosis, which was never observed in the absence of lymphoid hyperplasia. HGAL-mediated enhancement of BCR signalling may be important for efficient and timely completion of the GC reaction and selective activation of signalling pathways (for example, extracellular signal-regulated kinase and p38 but not Jun N-terminal kinases). Based on the presented mouse model, HGAL expression predisposes to lymphoid hyperplasia, polyclonal hypergammaglobulinemia and enhanced proliferation in response to BCR stimulation, culminating in systemic AA amyloidosis. B-lymphocytes in HGAL transgenic mice showed enhanced activation of Syk and RhoA signalling, suggesting this model recapitulates the biological effects of HGAL protein in human B cells. The observed polyclonal lymphoid hyperplasia was characterized by an accumulation of FO lymphocytes in the absence of GC lymphocytes and terminally differentiated plasma cells. The FO B cells in the lymphoid hyperplasia exhibited transcriptional signatures characteristic to FO/MZ B cells and plasma cells and were accompanied by polyclonal hypergammaglobulinemia in the absence of mature plasma cells, suggesting a block in terminal plasma cell differentiation whose nature is currently unknown. Studies examining HGAL’s effects on transcriptional signatures in human B cells are ongoing. In addition, whether the observed phenotype was due to expression of HGAL in the transgenic lines starting from progenitor and not specifically in the GC cells will need to be addressed. B-cell activation in the Sca1-HGAL mice led to reactive systemic AA amyloidosis not observed in the control animals. The molecular features and anatomical location of the observed amyloid deposits precisely recapitulated human AA amyloidosis complicating chronic inflammatory diseases (for example, rheumatoid arthritis). In these diseases reactive FO hyperplasia and lymphadenopathy are commonly observed [27] and frequently precede development of systemic amyloidosis. Heretofore, temporary AA amyloid deposits were induced in mice by exogenous agents (for example, casein, lipopolysaccharide), that would resolve without continued stimulation. Progressive and permanent AA amyloid deposits were observed in interleukin-6 and serum amyloid A activating factor 1 transgenic mice starting form 3–14 months of age [28] , [29] . In these models interleukin-6 and serum amyloid A activating factor directly stimulated serum amyloid A production, bypassing the preceding chronic inflammatory state observed in human disease. Conversely, HGAL mice develop AA amyloid deposits in a similar timeframe and show systemic lymphoid hyperplasia and hypergammaglobulinemia preceding amyloidosis onset, therefore, authentically recapitulating human amyloidosis associated with chronic inflammatory disorders. These mice may thus serve as an excellent model for this disease. The polyclonal lymphoid hyperplasia observed in the Sca1-HGAL mice were similar to the lymphoid hyperplasia detected in the BCL2 transgenic mice models, which also displayed polyclonal hypergammaglobulinemia. However, the mechanisms underlying these phenomena were different (increased cell proliferation and decreased apoptosis, respectively) [30] . Additional differences between these models are also noticeable. BCL2 transgenic mice develop lymphoid hyperplasia earlier than Sca1-HGAL mice, display autoimmune complex glomerulonephritis and a proportion of these animals develop lymphomas that were not detected in the Sca1-HGAL mice [30] , [31] , [32] , [33] . In contrast, infiltration of normal organs by B-lymphocytes and amyloidosis was observed only in the Sca1-HGAL mice. HGAL is expressed in the GC-derived B-cell lymphomas, but whether it has a role in lymphomagenesis is unknown. The Sca1-HGAL mice developed lymphoid hyperplasia, but not lymphomas. However, it is possible that HGAL may facilitate the transformation process. Gene expression arrays demonstrated significant overlap between genes upregulated in the lymphoid hyperplasia of the Sca1-HGAL mice and lymphomas driven by Bcl6/λMyc [24] . It is possible that the BCR-mediated proliferation detected in the Sca1-HGAL mice may cooperate with the antiapoptotic effects induced by BCL2 or differentiation arrest induced by BCL6 during the transformation process. Previous studies demonstrated similar cooperation between BCR and Myc in the genesis of B-cell lymphomas [34] . Use of the Sca1-HGAL mouse model to generate bitransgenic mice will help to elucidate the potential role of HGAL in lymphomagenesis. Mice and cell culture Human non-Hodgkin lymphoma cell lines Raji, VAL, BJAB and HBL-1 were grown as previously reported [35] . Human B-lymphocytes were isolated from healthy donor blood using EasySep Human B cell enrichment kit (StemCell Technologies, Vancouver, BC, Canada). A Sca1-HGAL plasmid in which HGAL cDNA is under the control of the mouse Ly-6E.1 promoter was generated as follows: the fragment containing the human HGAL-V5 cDNA, was inserted into the Cla I site of the pLy6 vector [15] , resulting in Sca1-HGAL vector. The transgene fragment ( Fig. 3a ) was excised from the vector by restriction digestion with Not I, purified for injection (2 ng μl −1 ) and injected into CBAxC57BL/6J fertilized eggs. Transgenic mice were identified by Southern analysis of tail snip DNA after Eco RI digestion. HGAL cDNA was used as a probe for detection of the transgene. The transgene copy number was determined by Southern blot analysis using copy standards prepared by mixing non-transgenic tail DNA with a known amount of transgene DNA as described in Camper [36] . A total of 47 and 28 animals derived from founder lines 102A and 102B, respectively, housed in pathogen-free conditions were used for the analyses. There were no differences between the founder lines. All animal experiments were performed in accordance with the guidelines of the Committees on Animal Research at University of Salamanca and University of Miami, and the National research Council. For cell sorter separation, B220 and CD22 lineage markers were used to purify cells from the spleen of both Sca1-HGAL or control wild-type mice by fluorescence-activated cell sorting (FACS) (FACSVANTAGE; Becton Dickinson). Purity of the sorted cells was over 98%, as determined by FACS reanalysis. Alternatively, mouse B-lymphocytes were isolated from mice spleen using EasySep mouse B-cell enrichment kit (StemCell Technologies). For analysis of B1 and B2 lymphocyte populations, single-cell suspensions were obtained from the spleens, LN, BM and peritoneal cavities of individual Sca1-HGAL and control mice. To obtain peritoneal cells, 6 ml of ice-cold PBS 1% fetal calf serum (FCS) were injected into the peritoneal cavity using a 25-g needle attached to a syringe. After injection, the peritoneum was gently massaged and cells were collected using a 5-ml syringe. Cells were washed with PBS 1% FCS and incubated for at least 5 min with CD16/CD32 Fc Block (clone 2.4G2) to minimize background staining. A total of 2 × 10 6 cells were stained for 30 min on ice with IgD-FITC (clone 11-26c.2a), CD5-PE (clone 53–7.3), Mac1-PerCP-Cy5.5 (clone M1/70) and IgM-APC (II/41) to identify the B2 and B1 cell subsets. All the antibodies were purchased from the BD Pharmingen. At least 1 × 10 5 cells were acquired using a BD C6 Accuri (BD Biosciences) and analysed by the Flowjo software (Tree Star). Antibodies, plasmids and chemicals, as well as procedures for cell tranfection, western blotting, immunoprecipitation, RhoA activity, GST pull-down and luciferase reporter assays are described in the Supplementary Methods . Flow cytometry and immunofluorescence microscopy Nucleated cells were obtained from total BM (flushing from the long bones), peripheral blood, thymus, LN and spleen. Contaminating red blood cells were lysed with RCLB lysis buffer and the remaining cells were then washed in PBS with 1% FCS. After staining, all cells were washed once in PBS with 1% FCS containing 2 mg ml −1 propidium iodide (PI) to allow dead cells to be excluded from both analyses and sorting procedures. The samples and the data were analysed in a FACSCalibur using CellQuest (Becton Dickinson) or FlowJo (Tree Star) software. Specific fluorescence of FITC, PE, PI and allophycocyanin excited at 488 nm (0.4 W) and 633 nm (30 mW), respectively, as well as known forward and orthogonal light scattering properties of mouse cells were used to establish gates. For each analysis a total of at least 50,000 viable (PI − ) cells were assessed. FACS definition of B-cell developmental stages was performed according to Kwon et al . [37] with minor modifications: BM pro-B cells (CD19 + c-Kit + ), BM pre-B cells (B220 + CD25 + IgM – ), BM immature B-cells (B220 + IgM hi IgD − ), BM recirculating B-cells (B220 + IgD hi ), peripheral transitional B-cells (B220 + IgM hi IgD hi ), peripheral mature-B cells (B220 + IgM lo IgD hi ), MZ B cells (B220 + CD21 hi CD23 lo ), FO B cells (B220 + CD21 int CD23 hi ). The subcellular localization of HGAL and Syk was assessed by stimulated emission depletion fluorescence nanoscope images [38] , as described in detail in the Supplementary Methods , together with the methodology for the immunohistochemistry and analysis of amyloid fibril protein. Gene expression analysis Using flow cytometry, CD22+B220+ splenocytes from adult Sca1-HGAL mice with hyperplastic follicles and wild-type littermates (four samples each) were sorted to ~98% purity, and profiled the corresponding gene expression patterns using Affymetrix GeneChip Mouse Gene 1.0 ST Arrays. Raw array microarray data files were submitted to GEO and are available under the accession number GSE35400. For probeset summarization, microarray CEL data files were subjected to a custom Chip Definition File (MoGene10stv1_Mm_ENTREZG_13.0.0) with a mapping of probes to Entrez Gene Identifiers as previously described [39] . Gene level data were normalized using robust multichip average within the BioConductor environment [40] . Significance analysis of microarrays [21] at a 10% FDR was used to identify the probe sets with significant differential expression between experimental conditions. We used DAVID [41] , Ingenuity Pathway Analysis tools (IPA 9/2011 Release), and the Molecular Signatures Database (MSigDB, v3.0) [42] , to assess whether differentially expressed genes show functional enrichment. For assessment of differentiation state, normal murine B-cell differentiation state signatures corresponding to Pro-B/Pre-B, transitional, FO/MZ, GC, plasmablast and plasma cell stages of differentiation were used as previously defined [22] . Over-representation of differentiation states within Sca1-HGAL compared with control B cells was inferred by assessing comparative enrichment of normal differentiation state signatures using GSEA [42] . GSEA was performed using a weighted enrichment statistic, signal-to-noise ratio ranking metric, and corrected for multiple hypothesis testing using 10,000 permutations to provide a multiple hypothesis testing-corrected FDR q -value. Reciprocal analysis was performed in order to validate positive enrichments within Sca1-HGAL B cells. Therein, publicly available gene expression data of normal murine B-cell differentiation states (GSE26408) was used to probe for enrichment of HGAL-induced genes within the FO/MZ and plasma cell differentiation states compared with all other differentiation states (1-versus-all analysis) using GSEA. Statistical analysis To test the differences in responses between cells, we used the two-way analysis of variance test for ex vivo B-cell proliferation assay and two-tailed Student’s t -test for remaining experiments. Mice survival curves were estimated using the product-limit method of Kaplan–Meier and were compared using the log-rank test. P -values <0.05 were considered statistically significant. How to cite this article: Romero-Camarero, I. et al . Germinal centre protein HGAL promotes lymphoid hyperplasia and amyloidosis via BCR-mediated Syk activation. Nat. Commun. 4:1338 doi: 10.1038/ncomms2334 (2013).